Orbitofrontal and striatal circuits dynamically encode the shift between goal-directed and habitual actions Shifting between goal-directed and habitual actions allows for efficient and flexible decision making. Here we demonstrate a novel, within-subject instrumental lever-pressing paradigm, in which mice shift between goal-directed and habitual actions. We identify a role for orbitofrontal cortex (OFC) in actions following outcome revaluation, and confirm that dorsal medial (DMS) and lateral striatum (DLS) mediate different action strategies. Simultaneous in vivo recordings of OFC, DMS and DLS neuronal ensembles during shifting reveal that the same neurons display different activities depending on whether presses are goal-directed or habitual, with DMS and OFC becoming more and DLS less engaged during goal-directed actions. Importantly, the magnitude of neural activity changes in OFC following changes in outcome value positively correlates with the level of goal-directed behavior. Chemogenetic inhibition of OFC disrupts goal-directed actions, whereas optogenetic activation of OFC specifically increases goal-directed pressing. These results also reveal a role for OFC in action revaluation, which has implications for understanding compulsive behavior. We often perform a similar action for different reasons, either to achieve a particular goal at that moment or because this action has been routinely reinforced and is now habitual [1] , [2] , [3] , [4] . Although the development of habits and rules is important for responding rapidly and accurately given a particular stimulus or state, we also encounter circumstances that make us re-evaluate the consequences of our actions. An inability to shift between habits and goal-directed actions (‘break habits’) may underlie distorted behaviours observed in obsessive compulsive disorder, addiction and other decision-making disorders [2] , [3] , [5] , [6] , [7] , [8] , [9] , [10] , [11] . The neural mechanisms and circuits governing the shift between these two behavioural strategies remain elusive. In the dorsal striatum, which receives vast inputs from most cortices [12] , [13] , [14] , the dorsal medial striatum (DMS) is necessary for goal-directed actions; lesions or inactivation of DMS render actions habitual instead of goal-directed [15] . Conversely, the dorsal lateral striatum (DLS) is necessary for habitual actions; lesions or temporary inactivation of DLS bias behaviour towards goal-directed actions [16] , [17] . Furthermore, the balance between habits and goal-directed behaviour is impaired in diseases such as obsessive-compulsive disorder [8] , in which the orbital frontal cortex (OFC) is dysfunctional [18] , [19] , [20] . This suggests that shifting between goal-directed and habitual actions could involve dynamic interactions between the corticostriatal circuits that underlie these individual behavioural strategies. However, how behavioural shifting is implemented is unknown. One possibility would be that these action strategies are encoded by different neuron ensembles in corticostriatal circuits, and a shift in behaviour would correspond to a shift of activity between neurons controlling goal-directed actions and neurons controlling habits. Another possibility would be that action strategies are concurrently encoded in the same neuronal ensembles in these circuits, and a shift between goal-directed actions and habits would correspond to a shift of activity in the same neurons as the different circuits compete to gain control over behaviour output. To disambiguate between these possibilities, we demonstrate a novel instrumental task where the same mouse would readily shift between performing a similar action for the same reward using either a goal-directed or a habitual strategy. Our results from experiments using functional lesions, in vivo recordings during action learning and revaluation, chemogenetic as well as optogenetic stimulations, suggest that shifts in activity of the same corticostriatal neuronal ensembles correspond to and can cause shifts between goal-directed and habitual actions. Mice readily shift between goal-directed actions and habits Paradigms to examine isolated goal-directed and habitual actions have been developed in humans and rodents, and outcome revaluation procedures examining control by the current expected value are commonly used to operationally distinguish these two behavioural strategies [10] , [11] . We designed a novel self-paced instrumental task in which individual mice readily shifted between performing goal-directed actions and habits. We took advantage of different contextual cues to differentiate between commonly used random ratio (RR) and random interval (RI) reinforcement schedules that bias towards the generation of goal-directed versus habitual actions, respectively [1] , [2] , [4] , [10] , [21] (Methods). We trained mice to press the same manipuladum (a lever placed in the same location) for the same reinforcer, using both RI and RR schedules of reinforcement ( Fig. 1a , Methods). Mice were initially trained to lever press on a continuous reinforcement (CRF) schedule, with the potential to earn 5, 15 and 30 rewards across 3 days. Then, mice underwent 2 days of RI30 (reinforcement follows the first press after an average of 30 s have passed) and RR10 (reinforcement follows on average the 10th lever press) training, followed by 4 days of RI60 and RR20 training. 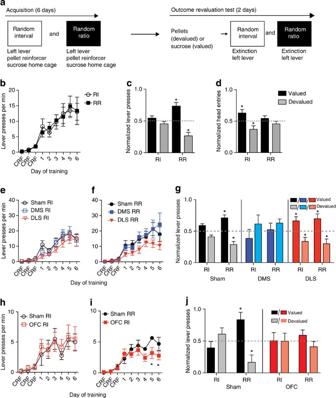Figure 1: Shifting between goal-directed and habitual actions. (a) Schematic of the within-subject behavioural design. Each day mice were trained to press the same manipulandum (identical lever in same position) for the same reinforcer on an RI schedule in one context, and on an RR schedule in a separate context. A control reinforcer was presented later in their home cages. After acquisition, mice were given a sensory-specific outcome revaluation test, in which they could free feed on either the control (valued state) or the previously earned reinforcer (devalued state). Mice were then immediately placed into one followed by the other training context for 5 min and non-reinforced lever presses were measured. (b) Average lever-presses per min across CRF and concurrent RI and RR schedule training for C57BL/6J mice (n=10). (c,d) Subsequent average lever presses (c) and head entries (d) (normalized to Revaluation state) made in RI and RR training contexts in Valued and Devalued states. (e,f,h,i) Average lever presses per min across CRF and concurrent RI and RR schedule training for Sham- (n=9), DMS- (n=5) and DLS (n=7)-lesioned mice (e,f) and for Sham (n=7) and OFC (n=5)-lesioned mice (h,i). (g,j) Average normalized to Revaluation state lever presses made in RI and RR training contexts during Valued and Devalued states for Sham-, DMS- and DLS-lesioned mice, (g) and Sham and OFC-lesioned mice (j). Repeated-measures ANOVA and one-way samplet-tests were used. Error bars indicate s.e.m. *P<0.05. (See alsoSupplementary Figs S1–4). Figure 1: Shifting between goal-directed and habitual actions. ( a ) Schematic of the within-subject behavioural design. Each day mice were trained to press the same manipulandum (identical lever in same position) for the same reinforcer on an RI schedule in one context, and on an RR schedule in a separate context. A control reinforcer was presented later in their home cages. After acquisition, mice were given a sensory-specific outcome revaluation test, in which they could free feed on either the control (valued state) or the previously earned reinforcer (devalued state). Mice were then immediately placed into one followed by the other training context for 5 min and non-reinforced lever presses were measured. ( b ) Average lever-presses per min across CRF and concurrent RI and RR schedule training for C57BL/6J mice ( n =10). ( c , d ) Subsequent average lever presses ( c ) and head entries ( d ) (normalized to Revaluation state) made in RI and RR training contexts in Valued and Devalued states. ( e , f , h , i ) Average lever presses per min across CRF and concurrent RI and RR schedule training for Sham- ( n =9), DMS- ( n =5) and DLS ( n =7)-lesioned mice ( e , f ) and for Sham ( n =7) and OFC ( n =5)-lesioned mice ( h , i ). ( g , j ) Average normalized to Revaluation state lever presses made in RI and RR training contexts during Valued and Devalued states for Sham-, DMS- and DLS-lesioned mice, ( g ) and Sham and OFC-lesioned mice ( j ). Repeated-measures ANOVA and one-way sample t- tests were used. Error bars indicate s.e.m. * P <0.05. (See also Supplementary Figs S1–4 ). Full size image Mice ( n =10) similarly increased the pressing rate across days of training in both schedules (main effect Training day: F8, 144=20.15, P <0.001), with mice making slightly more lever presses during RR training (interaction and main effects: Fs’ >3.2, ps’ <0.01) (Day 3 and 5 Bonferroni-corrected ps’ <0.05, Fig. 1b , Supplementary Fig. S1a ). Importantly, mice earned similar numbers of rewards, earned rewards at a similar rate and made a similar number of head entries into the food port between RI and RR schedule training (no interaction or Schedule main effect Fs’ <0.9, ps’ >0.05; main effect Training day: Fs’>2.40, ps ’<0.05) ( Supplementary Fig. S1b–d ). We also verified that in RI schedule training, there was no scalloping in responding [22] ( Supplementary Fig. S1g,h ). Further, we verified that the distribution of inter-reward intervals was the same between RI and RR schedules ( Supplementary Fig. S1i, j ), together suggesting that RI and RR schedules produced very similar patterns of lever-pressing behaviour. As the action strategy employed (goal-directed or habitual) cannot be elucidated during training [23] , we probed the degree to which an action in each training context was goal-directed or habitual during a brief (5 min) outcome revaluation test. We measured the number of non-reinforced lever presses in each context following sensory-specific satiation with either the outcome earned by lever pressing (devalued state) or a control outcome given daily in the home-cage (valued state) (Methods). We observed that mice reduced lever pressing only in the RR context, but not in the RI context following outcome revaluation (Repeated-measures analysis of variance (ANOVA) (Revaluation state × Schedule) interaction: F1, 18=4.51, P <0.05) (RR context: Bonferroni-corrected P <0.001) ( Fig. 1c ) ( Supplementary Fig. S1e ). Further one-sample t- tests of normalized lever pressing against chance 0.5 showed that only in the RR context did lever pressing significantly differ, with more pressing in the valued state, and less pressing in the devalued state (RR context: ts’ 9 >4.29, ps’ <0.002; RI context: ts’ <1.27, ps’ >0.2). These data show that lever pressing in the same mouse was sensitive to outcome revaluation in the RR but not in the RI schedule training context, and indicate that contextual information can induce mice to readily shift between executing a similar action in a goal-directed versus habitual manner. Non-rewarded head entries to the food port reduced following outcome revaluation in both previously RI and RR trained contexts (main effect Revaluation state F1, 18=6.11, P <0.05) (RI context: ts’ 10 =2.33, ps’ <0.05) ( Fig. 2d ). 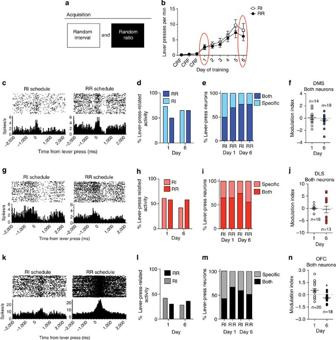Figure 2: Action encoding in different corticostriatal loops during RI and RR schedule training. (a) Schematic of the within-subject behavioural acquisition design and (b) rate of lever pressing under RI and RR schedules for recording mice (n=8). Example raster plots and peri-event time histograms (PETH) of the same DMS (c), DLS (g) and OFC (k) neurons showing lever-press-related activity under RI and RR reinforcement schedules on Day 6 of training. Each row in the raster is neural activity ±2 s around a lever press (time =0). Trials are sorted according to the order of lever presses made across the session. The percentage of lever-press-related activity per mouse during RI and RR schedule acquisition for DMS (d), DLS (h) and OFC (l). The percentage of lever-press-related neurons per mouse that change firing rate during lever-pressing behaviour in both RI and RR (Both-schedule neurons) or only during lever-pressing behaviour in RI or RR (Specific) in DMS (e), DLS (i) and OFC (m) across RI and RR acquisition. The modulation index for Both-schedule neurons across acquisition in DMS (f), DLS (j) and OFC (n).χ2-analyses, unpairedt-tests and one-samplet-tests were used. Error bars indicate s.e.m. *P<0.05. (See alsoSupplementary Figs S5–7). Figure 2: Action encoding in different corticostriatal loops during RI and RR schedule training. ( a ) Schematic of the within-subject behavioural acquisition design and ( b ) rate of lever pressing under RI and RR schedules for recording mice ( n =8). Example raster plots and peri-event time histograms (PETH) of the same DMS ( c ), DLS ( g ) and OFC ( k ) neurons showing lever-press-related activity under RI and RR reinforcement schedules on Day 6 of training. Each row in the raster is neural activity ±2 s around a lever press (time =0). Trials are sorted according to the order of lever presses made across the session. The percentage of lever-press-related activity per mouse during RI and RR schedule acquisition for DMS ( d ), DLS ( h ) and OFC ( l ). The percentage of lever-press-related neurons per mouse that change firing rate during lever-pressing behaviour in both RI and RR (Both-schedule neurons) or only during lever-pressing behaviour in RI or RR (Specific) in DMS ( e ), DLS ( i ) and OFC ( m ) across RI and RR acquisition. The modulation index for Both-schedule neurons across acquisition in DMS ( f ), DLS ( j ) and OFC ( n ). χ 2 -analyses, unpaired t- tests and one-sample t- tests were used. Error bars indicate s.e.m. * P <0.05. (See also Supplementary Figs S5–7 ). Full size image Corticostriatal circuits controlling action strategies We next examined the contribution of DMS and DLS to the shift between goal-directed and habitual actions. Excitotoxic lesions to either the DMS or DLS in mice (final n =5–9 per group) ( Supplementary Fig. S2a, Methods ) did not grossly impair the acquisition of lever-pressing behaviour under RI and RR schedule training (no interaction or Schedule main effect, main effect Training day: F16, 128=28.75, P <0.0001) ( Fig. 1e,f ) ( Supplementary Fig. S3b–d ). During outcome revaluation testing, sham mice reduced responding in the RR but not in RI contexts following outcome revaluation (Schedule × Revaluation state interaction: F1, 12=2.94, P =0.07; RR context Bonferroni-corrected P <0.01) (no main effects) (one-sample t- test (0.5) Valued and Devalued states: RI context: ts’ 8 <1.27, ps’ =0.06; RR context: ts’ 8 <4.45, ps’ <0.002) ( Fig. 1g ). However, during testing, we found that DMS-lesioned mice were always habitual and insensitive to outcome revaluation in both training contexts (Schedule × Revaluation state, no interaction or main effects: Fs’<0.95, ps’ >0.1) (one-sample t -test (0.5) on Valued and Devalued states: RI and RR contexts ts’ 4 <0.80, ps’ >0.4). Conversely, mice with DLS lesions reduced lever pressing following outcome revaluation, and were goal-directed in both training contexts (no interaction or main effect Schedule, main effect Revaluation state: F1, 10=11.29, P <0.01; RI and RR Schedule Bonferroni-corrected ps’ <0.01) (one-sample t- test (0.5) on Valued and Devalued states: RI and RR contexts ts’ 5 >2.53, ps’ <0.05) ( Fig. 1g , Supplementary Fig. S3g ). These results show that within-subject shifts are also controlled by dorsal striatal subregions [9] , [24] , and demonstrate that impediment to use the circuit involved in a particular action strategy results in a bias towards the use of the remaining intact circuit for action execution, suggestive of parallel encoding of both action strategies. As OFC has been implicated in various cue-related behaviours modulated by changes in expected value [25] , [26] , [27] , [28] , [29] , [30] , [31] , [32] , [33] , [34] , [35] , [36] , [37] , [38] , [39] , and OFC dysfunction has been linked to obsessive-compulsive disorder [18] , [19] , [20] , we examined its role in shifting between goal-directed and habitual actions. The OFC modulates medial striatum through direct projections [12] , [40] , [41] ( Supplementary Fig. S12b ) and indirectly through connexions with striatal projecting cortical areas, basolateral amygdala and ventral tegmental/substantia nigra ( pars compacta ) [12] ( Supplementary Fig. S12c,d ), nuclei known to contribute to instrumental actions [42] , [43] , [44] . We examined behaviours only in mice with localized more lateral versus medial OFC lesions [45] not affecting neighbouring cortices (final sham n =7, OFC n =5 per group, excluded n =5 for extension of lesion to neighbouring regions) ( Supplementary Fig. S2b ). OFC lesions did not affect the acquisition of lever-pressing behaviour in the RI schedule (Training day × Lesion group, no interaction or main effect Lesion group, main effect Training day: F8, 56=10.69, P <0.001) ( Fig. 1h,i , Supplementary Fig. S4b , although there was reduced response rate and fewer lever presses on the last 2 days of RR schedule training (Fs’>1.89, ps ’<0.08; Bonferroni corrected ps ’<0.05). Although visual inspection of the data suggested that mice with OFC lesions had higher response rates under RI than RR schedules, this was nonsignificant (F<1.04, P >0.4). Further, no effects of OFC lesion were observed on the number of rewards earned, rate of rewards earned or head entry behaviour in either schedules (no interaction or Lesion group main effect) (main effect Training day: Fs’ >1.96, ps’ <0.06) ( Supplementary Fig. S4c–e ). OFC-lesioned mice did not reduce lever pressing in either context following outcome revaluation (no interaction Schedule × Devaluation state, or main effects: Fs’<0.50, ps’ >0.05) (one-sample t- test (0.5) on Valued and Devalued states: RI and RR contexts: ts’ 4 <1.09, ps’ >0.3), whereas Sham mice shifted between habitual and goal-directed actions (Schedule × Devaluation state interaction: F1, 8=8.53, P <0.05) (Sham RR context: Bonferroni-corrected P <0.01) (one-sample t- test on Valued and Devalued states: RI context ts’ 6 =1.09, ps’ <0.35; RR context ts’ 6 >3.90, ps’ <0.05) ( Fig. 1j , Supplementary Fig. S4f ). Similar consumption between groups suggested no difference in outcome valuation ( Supplementary Fig. S4h ). Further, the impairment observed in OFC-lesioned mice was not caused by an inability to discriminate between contexts. Separate groups of OFC-lesioned mice trained independently on either RI ( n =10) or RR ( n =11) schedule of reinforcement (Methods) [46] , [47] still showed intact habitual actions ( Supplementary Fig. S4i–o ) but disrupted goal-directed actions ( Supplementary Fig. S4p–v ). There was no correlation between the response rate or reinforcement rate on the last day of training and the revaluation indices (Methods) for each mouse in either OFC-lesioned (rs’ 33 <0.13) or Sham mice (rs’ 26 <0.16). Together, this suggests that OFC is critical for the sensitivity of instrumental actions to changes in outcome value. Concurrent encoding of goal-directed and habitual actions Using multisite, multielectrode recordings in vivo (Methods, Supplementary Fig. S5g–k ), we recorded the activity of the same DMS, DLS and OFC neurons in each mouse during both RI and RR schedule training ( n =8 mice; Fig. 2a,b ) ( Supplementary Fig. S5 ). Recorded neurons showed similar baseline firing rates between training contexts ( Supplementary Fig. S6a,b,e,f,i,j ). As in other studies, we found evidence of changes in firing rate of DMS, DLS and OFC neurons around the lever press [47] (±2 s) during both RI and RR schedule training ( Fig. 2c,g,k ), with phasic increases in activity typically preceding lever pressing ( Supplementary Fig. S5i–k ). Previous findings using a cued task have suggested similar engagement of DMS and DLS circuits [48] , [49] . Using training schedules to directly bias the generation of instrumental habitual or goal-directed actions, we observed similar proportions of lever-press-related neurons between RI and RR schedules in DMS and DLS, as well as OFC circuits (per mouse, Fig. 2d,h,l ) ( ps’ >0.05). Further, we observed fairly similar proportions of up- and down-modulated neurons that increased or decreased their firing rate, respectively, during lever-press behaviour, ( Supplementary Fig. S7 ). In the within-subject design, we can examine activity changes in the same neuron during lever-pressing behaviour under schedules biasing goal-directed and habitual actions. Changes in lever-press-related activity could represent the same neuron-modulating activity under both RI and RR schedules (Both-schedule neurons), or Schedule-specific neurons that modulate their activity specifically during pressing in either the RI or the RR training context. We found a larger proportion of Both-schedule neurons than Schedule-specific neurons in DMS, DLS and OFC during RI and RR schedule training (DMS χ 2 =22.60, P <0.0001; DLS χ 2 =7.12, P =0.07; OFC χ 2 =13.49, P <0.004) ( Fig. 2e,i,m ). Given this finding, it could be that the same neurons (Both-schedule neurons) show different rate modulation during lever pressing, depending on the training schedule. We used a modulation index to examine the degree to which each Both-schedule neuron was differentially modulated during lever pressing under RR and RI schedules ( Supplementary Fig. S6c,g,i ), [(RR modulation rate−RI modulation rate)/(RR modulation rate+RI modulation rate)]. We found evidence in all three areas that some Both-schedule neurons showed stronger modulation in one or the other context (RI versus RR) ( Fig. 2f,j,n ). Averaging across Both-schedule neurons in DMS and DLS did not reveal modulation differences between RR and RI schedules; however, there was a training-induced shift in OFC modulation from Days 1–6 ( t 36 =3.66, P <0.001), with initially greater modulation in RR on Day 1 ( t 19 =2.54, P <0.05) to greater modulation in RI on Day 6 ( t 17 =3.3, P <0.01). Careful inspection of the index for DLS Both-schedule neurons revealed two distinct populations on Day 6, and analyses showed a non-Gaussian distribution on Day 6 (K2=6.04, P <0.05) ( Fig. 2j ). DLS Both-schedule neurons that increased firing rate during lever pressing showed a negative modulation index score (−4.41±0.76, t 5 =5.82, P <0.01). DLS Both-schedule neurons that decreased firing rate during lever-pressing behaviour showed a positive index score (4.65±0.34, t 6 =13.70, P <0.001). This suggests that DLS neurons become more inhibited with continued goal-directed training and more active during continued habit training. Shifts in neural modulation correspond to shifts in behaviour The findings presented above support the hypothesis that acquisition of goal-directed and habitual actions occurs in parallel in these circuits, and that often the same neurons are involved in both types of action, albeit differently modulated. This raises the possibility that the shift between goal-directed and habitual actions is reflected in differences in the modulation of Both-schedule neurons. To test this hypothesis, we examined the lever-press-related change in firing rates in DMS, DLS and OFC neurons during outcome revaluation testing ( Fig. 3a,b and Fig. 4a,b ) ( Supplementary Fig. S8 ) ( n =6 mice) (Schedule × Revaluation state interaction: F1, 28=6.36, P <0.05) (RR context: Bonferroni-corrected P <0.001) (RI context: P >0.05) (one-sample test (0.5) for Valued and Devalued states: RI context: ts’ 7 <0.24, ps’ >0.8; RR context: ts’ 7 >3.07, ps’ <0.05). Whereas normally goal-directed and habitual processes most likely contribute jointly to action control, outcome revaluation procedures promote goal-directed actions and habits to compete for action control [10] . 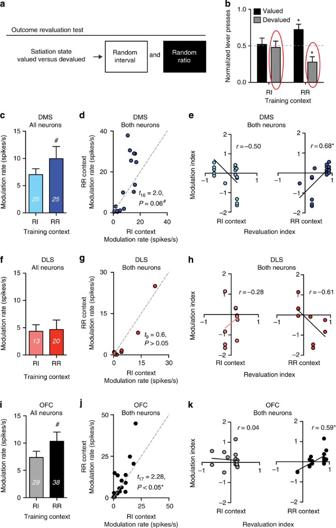Figure 3: Devalued state encoding of goal-directed and habitual actions in corticostriatal circuits. (a) Schematic of the within-subject outcome revaluation testing, and (b) normalized lever pressing on Valued and Devalued days in previously RI- and RR-trained contexts. Modulation rate (absolute change in firing rate) of lever-press-related DMS (c), DLS (f) and OFC (i) neurons (number in bar graph =nof modulated recorded neurons) during lever-pressing behaviour in previously trained RI and RR contexts in the Devalued state. X–Y scatter-plots of Both-schedule neuron modulation during lever-pressing behaviour in RI versus RR contexts in DMS (d), DLS (g) and OFC (j) in the Devalued state. Correlations between the modulation index of Both-schedule neurons in the Devalued state and the revaluation index for mice in RI and RR contexts for DMS (e), DLS (h) and OFC (k) Both-schedule neurons. Repeated-measures ANOVA, one-sample, unpaired and pairedt-tests, and Pearson correlation analyses were used. Error bars indicate s.e.m. *P<0.05. (See alsoSupplementary Figs S8 and S9).#P<0.09. Figure 3: Devalued state encoding of goal-directed and habitual actions in corticostriatal circuits. ( a ) Schematic of the within-subject outcome revaluation testing, and ( b ) normalized lever pressing on Valued and Devalued days in previously RI- and RR-trained contexts. Modulation rate (absolute change in firing rate) of lever-press-related DMS ( c ), DLS ( f ) and OFC ( i ) neurons (number in bar graph = n of modulated recorded neurons) during lever-pressing behaviour in previously trained RI and RR contexts in the Devalued state. X–Y scatter-plots of Both-schedule neuron modulation during lever-pressing behaviour in RI versus RR contexts in DMS ( d ), DLS ( g ) and OFC ( j ) in the Devalued state. Correlations between the modulation index of Both-schedule neurons in the Devalued state and the revaluation index for mice in RI and RR contexts for DMS ( e ), DLS ( h ) and OFC ( k ) Both-schedule neurons. Repeated-measures ANOVA, one-sample, unpaired and paired t- tests, and Pearson correlation analyses were used. Error bars indicate s.e.m. * P <0.05. (See also Supplementary Figs S8 and S9 ). # P <0.09. 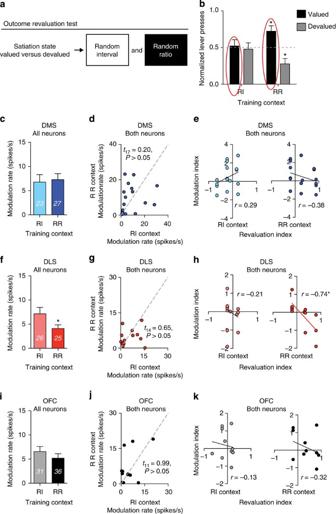Figure 4: Valued state encoding of goal-directed and habitual actions in corticostriatal circuits. (a) Schematic of the within-subject outcome revaluation testing, and (b) normalized lever pressing on Valued and Devalued days in previously RI- and RR-trained contexts. Modulation rate (absolute change in firing rate) of lever-press-related DMS (c), DLS (f) and OFC (i) neurons (number in bar graph =nof recorded modulated neurons) during lever-pressing behaviour in previously trained RI and RR contexts in the Valued state. X–Y scatter-plots of Both-schedule neuron modulation during lever-pressing behaviour in RI versus RR contexts in DMS (d), DLS (g) and OFC (j) in the Valued state. Correlations between the modulation index of Both-schedule neurons in the Valued state and the revaluation index for mice in RI and RR contexts for DMS (e), DLS (h) and OFC (k) Both-schedule neurons. Repeated-measures ANOVA, one-sample, unpaired and pairedt-tests, and Pearson correlation analyses were used. Error bars indicate s.e.m. *P<0.05. (See alsoSupplementary Figs S8 and S9). Full size image Figure 4: Valued state encoding of goal-directed and habitual actions in corticostriatal circuits. ( a ) Schematic of the within-subject outcome revaluation testing, and ( b ) normalized lever pressing on Valued and Devalued days in previously RI- and RR-trained contexts. Modulation rate (absolute change in firing rate) of lever-press-related DMS ( c ), DLS ( f ) and OFC ( i ) neurons (number in bar graph = n of recorded modulated neurons) during lever-pressing behaviour in previously trained RI and RR contexts in the Valued state. X–Y scatter-plots of Both-schedule neuron modulation during lever-pressing behaviour in RI versus RR contexts in DMS ( d ), DLS ( g ) and OFC ( j ) in the Valued state. Correlations between the modulation index of Both-schedule neurons in the Valued state and the revaluation index for mice in RI and RR contexts for DMS ( e ), DLS ( h ) and OFC ( k ) Both-schedule neurons. Repeated-measures ANOVA, one-sample, unpaired and paired t- tests, and Pearson correlation analyses were used. Error bars indicate s.e.m. * P <0.05. (See also Supplementary Figs S8 and S9 ). Full size image We first investigated the absolute change in rate modulation in DMS, DLS and OFC neuron ensembles during lever-press behaviour following outcome revaluation ( Fig. 3c,f,i ). Overall, there was a trend in OFC and DMS towards greater rate modulation in the previously trained RR versus RI contexts ( Fig. 3d,j ) (OFC t 65 =2.77, P =0.07; DMS t 48 =1.78, P =0.09), but not in DLS ( t 30 =014, P =0.10) ( Fig. 3g ). To examine the contribution of changes in the firing rate of the same neuron to differences observed in modulation rate above, we next examined the modulation rate of Both-schedule neurons in these circuits ( Fig. 3g,j ). There was greater rate modulation in the previous RR-trained context of OFC Both-schedule neurons ( t 17 =2.28, P <0.05), and DMS Both-schedule neurons (although to a lesser extent, t 16 =2.0, P =0.06) ( Fig. 3d,j ). This was not observed for DLS Both-schedule neurons or for Schedule-specific neurons ( ps’ >0.05) ( Supplementary Fig. S9 ). Next, we examined whether these changes in rate modulation of Both-schedule neurons really reflect the shift in behaviour following outcome revaluation. We correlated the modulation index in the Devalued state, with a revaluation index assessing the sensitivity of lever-press behaviour to changes in value in previously trained RI and RR contexts. We found that, in the Devalued state, the relative modulation of Both-schedule neurons in DMS and OFC in the previously RR- versus RI-trained contexts, positively correlated with the degree of goal-directed behaviour ( Fig. 3e,k ). That is, in the devalued state, the stronger the modulation of the same DMS and OFC neurons was during pressing in RR versus RI, the more sensitive the goal-directed lever pressing was to changes in outcome value. Interestingly, the converse tendency was observed in DLS ( Fig. 3h ). However, no significant correlations were observed for habitual actions in the RI context in DMS, DLS or OFC. Additionally, we did not observe a similar relationship between DMS, DLS and OFC neurons specific to the RI or RR schedule and behaviour ( Supplementary Fig. S9 ). In contrast, we did not observe differences in the rate modulation of DMS and OFC neurons between RI and RR contexts in the valued state, in which action value remains high ( ps’ >0.1) ( Fig. 4b,c,f,i ). Moreover, DMS and OFC Both-schedule neuron ensembles showed a similar rate modulation between RI and RR contexts ( ps’ >0.1) ( Fig. 4d,j ), with no correlation between modulation index and sensitivity to outcome revaluation ( Fig. 4e,k ). However, when action value was high, DLS neuron ensembles showed less rate modulation in the RR than in the RI context ( Fig. 4f ) ( t 49 =1.98, P =0.05). Further, the less DLS Both-schedule neurons modulated firing rate in RR versus RI; the more sensitive lever pressing in the RR context was to outcome revaluation ( Fig. 4h ). Together, these findings suggest that the sensitivity of actions to changes in outcome value during goal-directed behaviour is related to stronger modulation of OFC and DMS neurons, and weaker modulation of DLS neurons, in the RR versus the RI contexts. OFC conveys information about changes in action value These findings raise the hypothesis that reductions in goal-directed actions from the Valued to the Devalued state are related to changes in the overall modulation of OFC, DMS and DLS for each subject. To examine this, we first calculated the change in neural ensemble modulation (Both-schedule and Specific-schedule neurons) between the Valued and Devalued states in OFC, DMS and DLS for each mouse, and for both the RI and RR contexts ( Supplementary Fig. S10 ). Next, we correlated this change in modulation between Valued and Devalued states with the sensitivity to outcome revaluation. A striking positive correlation was observed in OFC ( P =0.01) (less in DMS, P =0.08), revealing that larger differences in OFC neural ensemble modulation between value states corresponded to greater sensitivity of actions to changes in outcome value (in the RR context, Fig. 5a ); that is, for each mouse, less OFC modulation in the Devalued versus the Valued state correlated with a stronger reduction in pressing following devaluation. This was not observed for habitual actions (RI context) for any area ( Fig. 5b ). 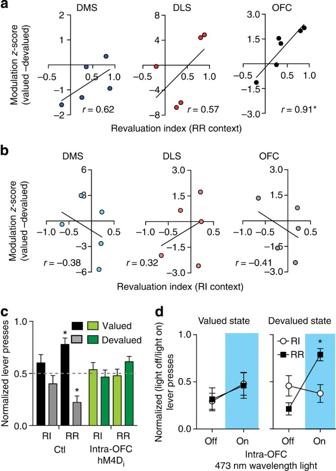Figure 5: OFC conveys information about changes in action value. Shift in OFC, DMS and DLS neural ensemble modulation between valued and devalued states for each mouse (changes inz-scores of lever-press-related modulation for Both-schedule and Schedule-specific neurons), correlated with the magnitude of goal-directed (a) and habitual behaviour (b) in the same animal as measured by a Revaluation index. (c) Effect of chemogenetic inhibition of OFC projection neurons on lever-press (normalized to Revaluation state) behaviour during outcome revaluation testing. Following either an OFC bilateral co-injection of cre-dependent hM4Direceptors and cre recombinase expressed under the CaMKIIα promoter (intra-OFC hM4Di:n=10) or cre-dependent hM4Diand a GFP virus (Ctl:n=11), mice were trained concurrently on RI and RR schedules using the within-subject design. On Valued and Devalued days, mice were given a systemic 1-h pretreatment with CNO (1 mg kg−1), and subsequent lever-press behaviour was recorded in each context. (d) Effect of bilateral optogenetic activation of OFC on lever-press (normalized to light on/off for each Revaluation state) behaviour during outcome revaluation testing. Following bilateral-OFC injection of ChR2-YFP expressed under the CamKIIα promoter and implantation of bilateral optic fibre ferrules, mice (n=6) were trained concurrently on RI (open circles) and RR (black squares) schedules using the within-subject design. On Valued and Devalued days, lever-press behaviour was recorded in each context for an initial 5 min without photostimulation, and during subsequent 5-min photostimulation with 10 hz, 5 ms pulses of 473 nm wavelength light. Repeated-measures ANOVA, one-sample, pairedt-tests, and Pearson’s correlation analyses were used. Error bars indicate s.e.m. *P<0.05. (See alsoSupplementary Figs S10–S12). Figure 5: OFC conveys information about changes in action value. Shift in OFC, DMS and DLS neural ensemble modulation between valued and devalued states for each mouse (changes in z -scores of lever-press-related modulation for Both-schedule and Schedule-specific neurons), correlated with the magnitude of goal-directed ( a ) and habitual behaviour ( b ) in the same animal as measured by a Revaluation index. ( c ) Effect of chemogenetic inhibition of OFC projection neurons on lever-press (normalized to Revaluation state) behaviour during outcome revaluation testing. Following either an OFC bilateral co-injection of cre-dependent hM4D i receptors and cre recombinase expressed under the CaMKIIα promoter (intra-OFC hM4D i : n= 10) or cre-dependent hM4D i and a GFP virus (Ctl: n =11), mice were trained concurrently on RI and RR schedules using the within-subject design. On Valued and Devalued days, mice were given a systemic 1-h pretreatment with CNO (1 mg kg −1 ), and subsequent lever-press behaviour was recorded in each context. ( d ) Effect of bilateral optogenetic activation of OFC on lever-press (normalized to light on/off for each Revaluation state) behaviour during outcome revaluation testing. Following bilateral-OFC injection of ChR2-YFP expressed under the CamKIIα promoter and implantation of bilateral optic fibre ferrules, mice ( n =6) were trained concurrently on RI (open circles) and RR (black squares) schedules using the within-subject design. On Valued and Devalued days, lever-press behaviour was recorded in each context for an initial 5 min without photostimulation, and during subsequent 5-min photostimulation with 10 hz, 5 ms pulses of 473 nm wavelength light. Repeated-measures ANOVA, one-sample, paired t- tests, and Pearson’s correlation analyses were used. Error bars indicate s.e.m. * P <0.05. (See also Supplementary Figs S10–S12 ). Full size image These results provide additional evidence suggesting that OFC ensembles are conveying information about action value. To test this hypothesis, we changed the activity of OFC projection neurons during outcome revaluation testing. We first reduced the activity of OFC projections using a chemogenetic approach with designer receptor exclusively activated by a designer drug (DREADD) clozapine N -oxide (CNO) [50] , [51] (Methods). A cre-dependent viral vector expressing G i -coupled hM4D i DREADD was bilaterally coinjected into OFC with either a virus expressing Cre recombinase under the control of the CaMKIIα promoter (restricting Cre expression to pyramidal cells) ( n =10; excluded n =2) or a control GFP virus (no DREADD expression) ( n =11) ( Supplementary Fig. S11 ). Mice trained concurrently on RI and RR schedules of reinforcement were given systemic injections of the synthetic agonist for hM4D i CNO (1 mg kg −1 ) 1 h prior to outcome revaluation testing, leading to a reduction in OFC activity ( Supplementary Fig. S11c,d ). Inhibition of OFC projection neurons via CNO activation of hM4D i receptors disrupted outcome revaluation in the RR context, with mice pressing similarly between valued and devalued states (no interaction or main effects: Fs’ <1.79, ps’ >0.1) (one-sample t- test (0.5) for Valued and Devalued states: RI and RR contexts: t s’ 9 <0.34, ps’ >0.05) ( Fig. 5c and Supplementary Fig. S11e ). As shown before, in control mice, devaluation resulted in a significant reduction in lever-press behaviour specifically in the RR context (Schedule × Revaluation state interaction: F1, 20=3.17, P =0.07; main effect Revaluation state: F1, 20=14.34, P <0.01) (RR context: Bonferroni-corrected P <0.01) (RI context: P >0.1) (one-sample t- test (0.5) for Valued and Devalued states: RI context: t s’ 10 <1.27, ps’ >0.2; RR context: t s’ 10 >4.55, ps’ <0.01), indicating that CNO administration had no effect on the shift between goal-directed and habitual actions in control mice. These findings suggest that reducing OFC projection neuron activity during outcome revaluation testing prevents changes in expected outcome value from influencing action performance. Next, we used an optogenetic approach to selectively activate OFC projection neurons during outcome revaluation testing ( Supplementary Fig. S12 ). As lesion, DREADD and in vivo recording data suggest that OFC activity is not involved in habitual actions, optogenetic activation of OFC projections should not have an impact on habitual actions. In contrast, lesions and DREAD-induced inactivation of OFC disrupted goal-directed actions and there was less OFC lever-press-related activity in the Devalued compared with the Valued state, suggesting that the reduced pressing observed following outcome devaluation in the RR context is related to this shift in OFC activity. This leads us to predict that optogenetic stimulation of OFC would increase pressing in the devalued state for goal-directed actions (in which action value is low) but not in the valued state (in which action value is high). Following injection of a virus expressing channelrhodopsin-2 under the control of the CaMKIIα promoter (restricting expression to pyramidal cells) [52] into OFC ( n =6) ( Supplementary Fig. S12a,e ), we concurrently trained mice on RI and RR schedules. We then optically stimulated OFC neurons in both contexts during outcome revaluation testing (that is, during both revaluation states) (5 ms pulses at 10 Hz) for 5 min (light-on), and compared the behaviour of the animals to 5 min of light-off in the same sessions. We found that in vivo bilateral stimulation of OFC projection neurons following a decrease in the outcome value was sufficient to increase lever pressing during this state (Devalued state (Light × Schedule): F1, 12=14.87, P <0.01) ( Fig. 5d ). Optogenetic stimulation of OFC did not increase pressing in the Valued state (Valued state F<0.03, P >0.05) ( Fig. 5d ) ( Supplementary Fig. S12f–k ), showing that this manipulation does not just increase the action of pressing, and suggesting that it does increase action value after devaluation. Furthermore, optogenetic stimulation did not alter habitual actions: photostimulation of OFC increased the frequency of lever pressing specifically in the RR context (biasing devalued conditions towards valuation, Bonferroni-corrected P <0.01) but not in the RI context ( P >0.05) ( Supplementary Fig. S12i–k ). These results confirm that changes in OFC activity are related to changes in the performance of goal-directed actions, and provide further evidence that OFC can convey information about action value. By investigating the activity of the same neurons in corticostriatal circuits as mice performed both goal-directed and habitual actions, we provide evidence that competing orbitofrontal and striatal circuits control context-induced shifts between habitual and goal-directed actions. We observed that the shifts in activity of the same orbitofrontal and dorsomedial striatal ensembles during outcome revaluation correlated with the degree of goal directedness, and strikingly, not with the execution of habits. These results suggest that, although during habitual actions neurons did change activity in relation to outcome revaluation, the behaviour of the animals was independent of the strength of this change. They also suggest that shifting back to goal-directed actions after habits are established corresponds to a dynamic shift in the activity of corticostriatal ensembles, as revealed by greater modulation of DMS and OFC, along with less modulation of DLS, during the performance of goal-directed pressing versus habitual responding. Finally, we observed that more lateral OFC is necessary for a shift to goal-directed actions following outcome revaluation. Our findings using lesions, recordings during outcome revaluation, and chemogenetic and optogenetic manipulations directly demonstrate a role for OFC in the balance between goal-directed actions and habits, and suggest that OFC may be conveying information related to action value. This contrasts with previous findings suggesting a stronger role for OFC in stimulus outcome relations than action–outcome relations [53] . One possibility is that the single action to single outcome design used here is more receptive to changes in action–outcome contingency [54] , hence allowing for a shift to habitual actions following disruptions to cortical circuits underlying goal-directed actions. It could also be that inhibiting a single action following devaluation recruits different neural mechanisms than the choice behaviour between two outcomes (albeit one devalued) observed following training with two actions and two outcomes. These results have important implications for understanding neuropsychiatric disorders where the balance between habits and goal-directed actions is disrupted, such as obsessive compulsive disorder [8] . It will be important to determine whether OFC use of outcome value to guide actions is through direct OFC projections to the dorsal striatum [12] , [39] , [40] , or through indirect projections, (for example, through OFC modulation of dopaminergic firing [36] during outcome revaluation). These findings are also important for understanding the execution of and the transition between goal-directed and habitual actions necessary for daily life, which are seemingly impaired in addiction and other decision-making disorders. Animals All experiments involved male C57Bl/6J mice at least 7 weeks of age (The Jackson Laboratory, Bar Harbour, ME, USA), and were approved by the National Institute on Alcohol Abuse and Alcoholism (NIAAA) and the NIAAA Animal Care and Use Committee, and were carried out in accordance with the NIH guidelines. Lesions A total of 0.2 μl of N-methyl-D-aspartic acid was infused at a rate of 60 nl min −1 (via Hamilton syringe) to induce excitotoxic lesions of the DMS (B: AP 0.5 mm, L±1.5 mm and V −2.5 mm from the skull) or DLS (B: AP 0.5 mm, L±2.65 mm and V −3.0 mm from the skull). Ibotenic acid 0.3 μl (10 mg ml −1 ) was infused (via pump, Razel, Scientific) (0.1 μl min −1 ) to induce excitotoxic lesions of the OFC (B: AP 2.7 mm, L±1.75 mm and V −2.25 mm from the dura). For Sham mice, injectors were lowered to the target site but no infusion was given. Mice were allowed to recover for at least 10 days before the start of behavioural procedures. Mice were perfused and the brains post-fixed with 4% w/v paraformaldehyde, with lesion placement identified through Nissl staining of 50-μm brain slices. Only mice with lesions located with DMS, DLS or OFC (see Supplementary Fig. S2 ) were included. (Final n ’s: Striatal Sham lesion=7, DMS lesion=5, DLS lesion=6; OFC Sham=8–10, OFC lesion=5–11). Chemogenetic inhibition of OFC For chemogenetic inhibition of OFC projection neurons, cre-inducible AAV-hSyn-DIO-hM4D i -mCherry (Gene Therapy Vector Core at the University of North Carolina) was infused bilaterally into OFC (same coordinates as above) with either AAV2/9. CamKII.HI.GFP-Cre or AAV2/9. GFP virus (University of Pennsylvania vector core) (100 nl per side for each virus). Three weeks following injection, hM4D i mice ( n =10) and control mice ( n =11) were trained on the within-subject design. During outcome revaluation testing, mice were given a 1-h pretreatment with CNO (1 mg kg −1 )(10 ml kg −1 ) before operant procedures. To confirm hM4Di activity, we implanted an electrode array at the site of virus infusion. Firing rate of OFC neurons was assessed 1 h after CNO injection relative to the preceding drug-free baseline-firing rate ( Supplementary Fig. S11 ). Virus spread was assessed under a fluorescence microscope. Optogenetic activation of OFC For optogenetic activation of OFC projection neurons, AAV2/9.CamKIIChR2-YFP [52] (Standford-Deisseroth lab) (200–300 nl per side) was infused bilaterally into OFC (same coordinates as above) and bilateral optic fibre ferrules were implanted (V −2.35 mm from the dura) in OFC. Five weeks following injections, mice ( n =6) were trained on the within-subject design. During outcome revaluation testing, after pre-feeding mice were lightly anesthetized (isoflurane) and connected with a ceramic sleeve to a 473-nm laser via fibre optic rotary joint to optical fibres (200 μm core diameter) that was controlled by a Master8 stimulator to deliver 5-ms pulses at 10 Hz (<5 mW power at the tip of the fibre). To confirm optogenetic activation of OFC neurons, in a subset of mice ( n =2), we attached a fibre optic ferrule to the side of an electrode array to record neural activity at the site of stimulation. We assessed light activation of OFC neurons in both anesthetized and awake-behaving preparations ( Supplementary Fig. S12 ). AAV2/9.CamKIIChR2-YFP spread and ferrule placement were assessed under a fluorescence microscope. Behavioural procedures Mice were placed in operant chambers in sound-attenuating boxes (Med-Associates, St Albans, VT) in which they pressed a single lever (left or right) for an outcome of either regular ‘chow’ pellets (20 mg pellet per reinforcer, Bio-Serve formula F05684) or sucrose solution (20–30 μl of 20% solution per reinforcer). The other outcome was provided later in their home cage and used as a control for general satiation in the revaluation test. Before the training commenced, mice were food restricted to 90% of their baseline weight, at which they were maintained for the duration of experimental procedures. For the within-subject design, training was conducted as follows: each day mice were trained in two separate operant chambers distinguished by contextual cues (black and white striped walls versus clear plexiglass). For each mouse, the order of schedule exposure, lever position and the outcome obtained upon lever press were kept constant across contexts. However, mice were counterbalanced for context, schedule order, lever position and the outcome earned. Each training session commenced with an illumination of the house light and lever extension, and ended following schedule completion or after 90 min with the lever retracting and the house light turning off. On the first day, mice were trained to approach the food magazine (no lever present) in each context on a random time (RT) schedule, with a reinforcer delivered on average every 60 s for a total of 15 min. Next, mice were trained in each context on CRF, where every lever press made was reinforced, with the possible number of earned reinforcers increasing across training days (CRF5, 15 and 30) (recording mice took on average 6±1 days of CRF training (CRF5, 15, 30 × 4). After acquiring lever-press behaviour, mice were trained on RI (RI30 2 days/RI60 4 days) and RR (RR10 2 days/RR20 4 days) schedules of reinforcement, with schedules differentiated by context, with the possibility of earning 15 reinforcers in each context or until 90 min had elapsed. Outcome revaluation testing occurred across two consecutive days as previously described ( 28 ). In brief, on the valued day, mice had ad libitum access to the home cage outcome for 1 h before serial brief non-reinforced test sessions in the previous RI and RR training contexts. On the devalued day, mice were given 1 h of ad libitum access to the outcome previously earned by lever press, and then underwent serial non-reinforced test sessions in each training context. The order of context exposure during testing was the same as training exposure, with the order of revaluation day counterbalanced across mice. Tests in each context were either 10 min (recording and ferrule mice) or 5 min (all lesion and DREADD mice) in duration. For mice in the between-schedule (RI or RR training) lesion experiment, training and devaluation testing proceeded exactly as for mice in the lesion experiment using the within-subject design (RI and RR), except that mice were only trained on the RR or RI schedule in one context [45] . Additionally, to equate the total number of possible reinforcers earned between lesion experiments, mice had the opportunity to earn 30 reinforcers or until 90 min had elapsed during the RI or RR training. In vivo extracellular recordings Mice were implanted with multi-electrode arrays for in vivo recordings of neural activity during awake behaviour [47] , [55] . Mice were implanted with two arrays, one targeting the OFC, and the other targeting the DMS and DLS. The array used in the OFC consisted of two rows of eight platinum-plated tungsten electrodes (35 μm, CD Neural), with electrodes spaced 150 μm apart, and rows 200 μm apart. For the OFC, arrays were centred A2.6 mm and L1.75 mm to Bregma, and V 2.25–2.4 mm from the surface of the brain. For the dorsal striatum, the array consisted of two rows of eight electrodes (platinum-coated tungsten, 50 μm, CD Neural), with electrodes spaced 200 μm apart and row spaced 1250 μm apart so that one row targeted the DMS and the other row targeted the DLS. For the dorsal striatum, arrays were centred A0.5 mm and L1.75 mm from Bregma and V 2.2–2.4 mm from the surface of the brain. Mice were perfused and brains fixed with 4% w/v paraformaldehyde, and array placement was verified using Nissl-stained brain slices (50 μm). Neural recordings during behaviour Mice were allowed at least 2 weeks of recovery before the start of behavioural and recording procedures. In brief, spike activity was recorded using the MAP system (Plexon Inc., TX) and initially sorted using an online-sorting algorithm. Mice were moved from one context to the other without disconnecting the headstage, and the same online-sorting algorithm was used in both contexts on the same day. TTL pulses were used to synchronize the recordings with the lever-press behaviour, to behaviourally timestamp the neural activity (10-ms resolution of the behaviour). Data were then resorted offline (Offline Sorter, Plexon Inc.) to identify single-unit neuronal activity based on waveform, amplitude and interspike-interval histogram (no spikes during a refractory period of 1.3 ms) [40] . For the dorsal striatum, in order to have mainly putative striatal medium spiny neurons in our analyses, units with a waveform trough half-width of <100 μs and baseline firing rate of >10 Hz, as well as those with a waveform trough half-width >250 μs were excluded [56] . In OFC, units clustered around an amplitude of 150 μV, waveform trough half-width of 200 μs and frequency of 3.5 Hz; in order to have mainly potential pyramidal neurons in our analyses, units with values two standard deviations greater than the population mean were excluded from the analyses. Lever-press-related neurons To examine task-related neural activity, for each previously isolated recorded unit we constructed a peri-event histogram (PETH) around time-stamped lever press and head entry events, in which neural activity was averaged in 20-ms bins, shifted by 1 ms and averaged across trials to analyse amplitude and latency during the recorded behaviours. Using the distribution of the PETH from 5,000–2,000 ms before the task as baseline activity, we slid 1-ms steps across 20-ms bins from 2,000 ms before to 2,000 ms after task-related events. A task-related neuron was up-modulated if it had a significant increase in firing rate defined as at least 20 consecutive overlapping bins, with a firing rate larger than a threshold of 99% above baseline activity. A task-related neuron was down-modulated if it had a significant decrease in firing rate of at least 20 consecutive bins had a firing rate smaller than a threshold of 95% below baseline activity [47] , [56] . The onset of task-related activity was defined as the first of these 20 consecutive significant bins. Schedule-specific neurons were units that only showed a significant up-or down-modulation in the PETH around the behavioural event in the RI or RR context. Both-specific neurons were units that showed a significant up- or down-modulation in the PETH around the behavioural event in both RI and RR contexts. Rate modulation was defined as maximum or minimum firing rate in the time window from the beginning to the end of the consecutive significant bins minus baseline. The same analyses performed using a less conservative window of 1,000 ms before and after task events did not alter the present findings. See example average frequency traces ( Fig. 2c,g and k ). Statistical analyses The α level was set at 0.05 for all analyses performed, except otherwise indicated. Initial analyses showed normal distributions for all behavioural data. All behavioural analyses and in vivo rate modulation data were analysed using paired and unpaired t- tests, as well as two-way and repeated measure ANOVAs with post-hoc analyses performed using Bonferroni-corrected paired t- tests where appropriate, including normalized lever presses during outcome revaluation (normalization: (lever presses for Valued or Devalued states/total lever presses Valued+Devalued states)). We also included one-sample t- tests for normalized data to examine whether each condition differed from chance (0.5); that is, normalized data produced a distribution of lever presses between Valued and Devalued states for each schedule, and value of 0.5 reflects the same level of lever pressing between Valued and Devalued states. χ 2 analyses were used to look at proportional differences in percentage of lever-press-related activity, direction of modulation and the contributions of Both versus Specific neurons to the above changes. Correlation analyses were performed using Pearson’s ( r ) correlation coefficient α =0.05 for all tests performed. Rate modulation values of lever-press-related activity were used to calculate the modulation index for each neuron ((RR rate modulation−RI rate modulation)/(RR rate modulation+RI rate modulation)). To investigate the shift in ensemble neural activity for each area in Figure 5a,b , we calculated the difference between devalued and valued days in average rate modulation z -score around the lever press for all lever-press-related neurons (Both and Specific) within an area for each subject in RI and RR contexts. To examine the degree of goal directedness during outcome revaluation ( Figs 3 , 4 , 5 ), we calculated a revaluation index ((lever presses valued state−lever presses devalued state)/(lever presses valued state+lever presses devalued state)) for each mouse for the RR and RI contexts. Correlation analyses were performed using Pearson’s ( r ) correlation coefficient α =0.05 for all tests performed. Data analyses were performed using Neuroexplorer, Graphpad Prism, and Matlab (Mathworks). How to cite this article: Gremel, C. M. et al. Orbitofrontal and striatal circuits dynamically encode the shift between goal-directed and habitual actions. Nat. Commun. 4:2264 doi: 10.1038/ncomms3264 (2013).